Controlling the influence of Auger recombination on the performance of quantum-dot light-emitting diodes Development of light-emitting diodes (LEDs) based on colloidal quantum dots is driven by attractive properties of these fluorophores such as spectrally narrow, tunable emission and facile processibility via solution-based methods. A current obstacle towards improved LED performance is an incomplete understanding of the roles of extrinsic factors, such as non-radiative recombination at surface defects, versus intrinsic processes, such as multicarrier Auger recombination or electron-hole separation due to applied electric field. Here we address this problem with studies that correlate the excited state dynamics of structurally engineered quantum dots with their emissive performance within LEDs. We find that because of significant charging of quantum dots with extra electrons, Auger recombination greatly impacts both LED efficiency and the onset of efficiency roll-off at high currents. Further, we demonstrate two specific approaches for mitigating this problem using heterostructured quantum dots, either by suppressing Auger decay through the introduction of an intermediate alloyed layer, or by using an additional shell that impedes electron transfer into the quantum dot to help balance electron and hole injection. Colloidal quantum dots (QDs) exhibit narrow-band, highly efficient and widely tunable emission. Further, they can be fabricated and processed via low-cost solution-based techniques compatible with lightweight, flexible substrates [1] . Owing to these features, QDs have been actively investigated for use in optoelectronic devices ranging from down-converters in backlit displays [2] , [3] and light-emitting diodes (LEDs) [4] , [5] , to lasers [6] , photodetectors [7] and solar cells [8] . Among these potential applications, the realization of high-performance electrically pumped QD-based LEDs (QD-LEDs) has been of particular interest due to its potentially immediate and significant impact in display and lighting technologies. Since the first demonstration of QD-LEDs [4] , there have been numerous attempts to improve the device performance by optimizing both the materials synthesis and the device architecture [9] , [10] , [11] , [12] , [13] , [14] , [15] , [16] , [17] . An impressive result of these efforts is the recent demonstration of QD-LEDs with performance exceeding that of fluorescent organic LED (OLEDs), which have been under intense investigation for at least two decades [11] , [12] , [13] . In recent years, the understanding of the physics underlying the operation of QD-LEDs, and specifically the factors that limit their performance, has greatly improved. However, the role of multicarrier effects including Auger recombination in QD-LEDs is still largely unclear. It has been established that in traditional quantum-well-based LEDs, Auger recombination is responsible for efficiency roll-off (also known as droop) at high-driving currents [18] , [19] . Some recent studies have suggested that a similar effect is also responsible for efficiency roll-off in QD-LEDs [9] . However, this view is not universally accepted, as other works have attributed it to the effect of the applied electric field, which leads to spatial separation between electrons and holes, and thus reduces the rate of radiative recombination due to reduced electron-hole overlap [20] , [21] . Here we analyse the role of Auger recombination in QD-LEDs by conducting a systematic characterization of device performance in conjunction with studies of the dynamics of photoexcited carriers directly within the device structure. In our LEDs, we use a series of structurally engineered core/shell QDs that are characterized by similar band gaps ( E g of ca. 2 eV) and valence/conduction-band positions, but distinctly different rates of non-radiative Auger recombination [22] . By correlating device performance with the photophysical properties of the QDs, we find that both LED efficiency and the onset for efficiency roll-off are strongly influenced by multicarrier dynamics. Specifically, time-resolved photoluminescence (PL) measurements indicate that a large contribution to QD emission originates from negatively charged excitons (that is, negative trions) that are formed as a result of an imbalance between electron and hole injection. We further show that device efficiency can be improved by use of either of two distinct types of specifically engineered heterostructured QDs. The first type of QDs features an alloyed core-shell interface, which leads to suppressed Auger recombination and increased emission efficiency of charged species. In the second, the conduction-band edge of the shell is intentionally raised in order to moderately impede electron injection and thus improve the charge-injection balance within the QD active layer. Use of either type of QDs enhances peak emission efficiency, and significantly increases the threshold current of efficiency roll-off. Structural and spectroscopic properties of QD emitters In our studies, we use an inverted LED design in which electrons are injected into QDs using an indium tin oxide (ITO) cathode coated with a 50-nm thick inorganic charge-transport layer (CTL) made of ZnO colloidal nanoparticles ( Fig. 1a ; see also Supplementary Fig. S1 for optical spectra of various device components). Holes are injected via an organic CTL made of 4,4′- bis ( N -carbazolyl)-1,1′-biphenyl (CBP, 60 nm) separated from an Al anode by a MoO x (10 nm) spacer. Sandwiched between the CTLs is the emitting layer of one-to-two monolayers of QDs. We have selected this LED architecture as a test platform for our studies for two major reasons. First, to date, this type of LED with hybrid inorganic/organic CTLs has offered the best overall performance by combining a low turn-on voltage and high device efficiency and brightness with good operational stability [11] , [12] , [13] , [14] , [15] . Second, unlike other types of QD-LEDs that utilize complex excitation mechanisms (for example, exciton injection via Förster-type transfer from one of the CTLs) [9] , [23] , these inverted LED structures rely on direct injection of charges into QDs from adjacent CTLs [11] , [12] , [13] , which allows us to more easily relate the results of our spectroscopic studies to the overall device performance in the regime of electrical injection. 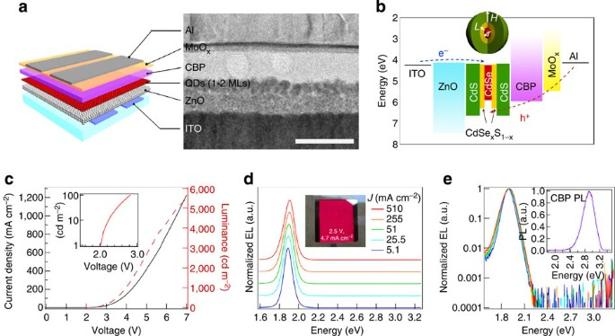Figure 1: Device structure, performance characteristics and emission spectra of a QD-LED. (a) Schematic illustration and cross-sectional TEM image (scale bar, 100 nm), and (b) energy band-diagram of a QD-LED with an inverted device architecture: ITO//ZnO nanoparticles (50 nm)//QDs (1–2 MLs)//CBP (60 nm)//MoOx(10 nm)//Al. (c) Current–voltage (J–V) and luminance-voltage (L–V) characteristics of a typical QD-LED studied in this work (inset: expandedL–Vcharacteristics showing the turn-on voltage,Von, of 2 V; (d) normalized EL spectra of the same device under varied current densities (Inset: photograph of a QD-LED with pixel area of 1.2 × 1.2 cm2under a 2.5 V bias;J=4.7 mA cm−2); (e) same as in ‘d’ with the EL intensity shown on a log scale to demonstrate the lack of any contribution of CBP emission to device EL (inset: a PL spectrum of CBP). Figure 1: Device structure, performance characteristics and emission spectra of a QD-LED. ( a ) Schematic illustration and cross-sectional TEM image (scale bar, 100 nm), and ( b ) energy band-diagram of a QD-LED with an inverted device architecture: ITO//ZnO nanoparticles (50 nm)//QDs (1–2 MLs)//CBP (60 nm)//MoO x (10 nm)//Al. ( c ) Current–voltage ( J – V ) and luminance-voltage ( L–V ) characteristics of a typical QD-LED studied in this work (inset: expanded L – V characteristics showing the turn-on voltage, V on , of 2 V; ( d ) normalized EL spectra of the same device under varied current densities (Inset: photograph of a QD-LED with pixel area of 1.2 × 1.2 cm 2 under a 2.5 V bias; J =4.7 mA cm −2 ); ( e ) same as in ‘ d ’ with the EL intensity shown on a log scale to demonstrate the lack of any contribution of CBP emission to device EL (inset: a PL spectrum of CBP). Full size image To probe the role of single-exciton versus multicarrier dynamics in QD-LEDs, we use a new class of structurally engineered CdSe/CdS core/shell (C/S) and CdSe/CdSe 0.5 S 0.5 /CdS core/alloy layer/shell (C/A/S) QDs [22] . Specifically, we fabricated a series of QD samples having the same CdSe core radius ( r =1.5 nm) and a varying thickness of the CdS shell ( H ); the thicknesses of the interfacial CdSe 0.5 S 0.5 alloy layer ( L ) in the C/A/S sample is 1.5 nm (see Supplementary Fig. S2 for transmission electron microscopy (TEM) images and optical spectra of QD samples). All of these samples have similar band-gap energy (~2 eV) and positions of conduction- and valence-band edges ( Fig. 1b ). Due to the small conduction-band offset between CdSe and CdS, the electron wavefunction in these QDs is delocalized over the entire core/shell structure, while the hole wavefunction is tightly confined to the core due to the large confinement-potential in the valence-band at the core/shell interface. Increasing the shell thickness leads to a reduction in the electron-hole overlap, which should result in a lengthening of single-exciton lifetimes ( τ X ). This trend is indeed observed experimentally ( Table 1 ): as the thickness of the shell in the C/S QDs is increased from 2.0 to 5.5 nm, τ x increases from 20 to 40 ns. Table 1 Photophysical properties of QDs and device characteristics of corresponding QD-LEDs. Full size table The negative-trion ( X − ) and biexciton ( XX ) lifetimes ( and τ XX , respectively) also become longer for C/S samples with thicker shells ( Table 1 ; see Methods section for details of the measurements). In QDs, charged exciton and bixciton decays are dominated by Auger recombination where the electron-hole recombination energy is transferred to a third charge carrier (an electron in the case of negative trions; an electron or a hole in the case of biexcitons). As indicated by numerous previous studies, Auger lifetimes scale linearly with the QD volume for simple, mono-component QDs [24] , [25] . This statement can be generalized for heterostructured QDs by considering the effective volumes occupied by the carriers involved in Auger recombination instead of simply total QD volume. For the C/S structures, delocalization of the electron wavefunction into the shell leads to a significant increase in the effective volume specifically of the electron, which is the main factor responsible in the C/S structures for the increase of and τ XX with increasing H [22] . The insertion of a 1.5-nm-thick CdSe x S 1−x alloy layer between the CdSe core and CdS shell does not have a significant effect on a single-exciton lifetime, but leads to an appreciable increase in both negative trion and biexciton lifetimes as compared with C/S QDs of the same volume (lines 3 and 4 in Table 1 ), indicating a reduction in the Auger decay rate. Interestingly, the larger relative change in biexciton lifetime is consistent with an even stronger suppression of the hole-mediated (or ‘positive trion’) Auger recombination. Previously, this suppression of Auger recombination in C/A/S QDs was attributed to a ‘smoothing’ of the core-shell interface potential [22] , which according to calculations [26] , [27] reduces the overlap between wavefunctions of the initial and the final states of the carrier excited in the course of Auger decay. Thus, the use of the C/S and C/A/S samples that exhibit similar single-exciton dynamics but distinctly different rates of Auger decay allows us to selectively probe the influence of multicarrier recombination on the performance of QD-LEDs. Effect of Auger decay suppression on QD-LED performance All QD-LEDs fabricated in the present study show p-n diode-like current-density ( J )-voltage ( V ) characteristics ( Fig. 1c ), with a turn-on voltage ( V on ) near the band-gap energy of the QDs ( Table 1 and Supplementary Fig. S3 ). This suggests that this device architecture results in highly efficient carrier injection from CTLs into QDs, and further that the structural variations within the series of studied QDs, and specifically the insertion of the interfacial alloy layer, does not have any appreciable effect on carrier injection efficiency. QD-LEDs display electroluminescence (EL) solely from QDs without any noticeable contribution from CTLs (CBP PL peaks at ~2.85 eV; inset of Fig. 1e ) for the range of current densities used in the present study (5 mA cm −2 ≤ J ≤510 mA cm −2 , Fig. 1d,e ; see also Supplementary Fig. S3 ). This indicates that QDs serve as the primary exciton recombination centres during device operation and further suggests that charge carrier leakage through the QD layer that might otherwise lead to parasitic emission from the CTLs is negligible. The use of the inverted architecture allows us to enhance charge injection into the QDs and achieve a significant improvement in device performance compared with previously reported LEDs employing the same type of C/S QDs but in a more traditional architecture (that is, with an ITO anode and a metal cathode) [28] . Specifically, our present structures exhibit the following set of operational parameters: V on =2.0 V, external quantum efficiency (EQE) of up to 1.8%, and maximum luminance of more than 7,000 cd m −2 . This compares favourably to the parameters of previously published devices, which were characterized by V on =3.0 V, EQE of up to 0.11%, and maximum luminance of ca . 1,000 cd m −2 . More importantly, the new devices reach high brightness and current densities under relatively low-applied biases: current densities in excess of 255 mA cm −2 and brightness greater than 2,000 cd m −2 can be realized at <6 V. This enables us to study device performance with high concentrations of carriers within QDs under conditions in which the influence of applied electric field [20] and/or joule heating on the QD emission efficiency is minimal. 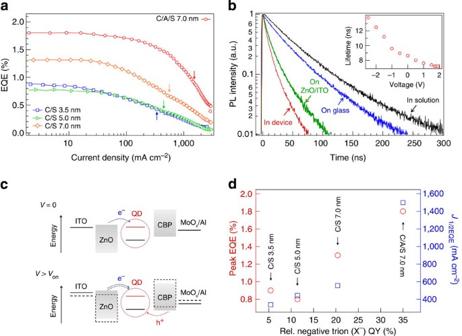Figure 2: Influence of QD charging on LED performance. (a) EQE versus current-density of QD-LEDs with different types of QDs. The onset of EQE roll-off (J1/2EQE, indicated by arrows) shifts to higher currents with increasing degree of suppression of Auger recombination. (b) PL decay dynamics of C/A/S QDs (total radius 7.0 nm; line 4 inTable 1) in solution (black), as a film on a glass substrate (blue), as a film on a ZnO/ITO substrate (green), and within a QD-LED at zero bias (V=0) (red). Inset: PL lifetime for QDs within the device as a function of applied voltage (V≤Von). (c) Schematic illustration of QD charging in QD-LEDs under zero bias (upper panel) and under operational conditions (V>Von; lower panel). (d) Peak EQE andJ1/2EQEof QD-LEDs as a function of a relative PL QY of a negative-trion (). Figure 2a displays the dependence of EQE on J during a current sweep. Regardless of the type of QDs incorporated into the LED, EQE stays approximately constant up to a current density of ( J =10 mA cm −2 ) and then gradually decreases at higher currents. Interestingly, there is no direct correlation between the value of the peak EQE and the solution PL quantum yield (QY) of the QD solutions within the series of studied samples ( Table 1 ). For instance, although the C/A/S 7.0 nm QDs and the C/S 7.0 nm QDs (lines 3 and 4 in Table 1 ) exhibit the lowest solution PL QYs, QD-LEDs based on these QDs yield higher peak EQEs than those of devices based on 3.5 and 5.0 nm C/S QDs (lines 1 and 2 in Table 1 ). This implies that even at low current, and hence low-exciton densities, the QD-LED efficiency is not solely dependent on single-exciton PL QY. This assessment is confirmed by the observation of an appreciable improvement in the EQE for the 7 nm C/A/S sample (1.8%) compared with the EQE of 7 nm C/S sample (1.3%), which occurs despite identical single-exciton PL QYs measured for solution samples and similar single-exciton lifetimes (lines 3 and 4 in Table 1 ). All of these observations suggest that factors other than single-exciton properties have a considerable effect on LED performance. Figure 2: Influence of QD charging on LED performance. ( a ) EQE versus current-density of QD-LEDs with different types of QDs. The onset of EQE roll-off ( J 1/2EQE , indicated by arrows) shifts to higher currents with increasing degree of suppression of Auger recombination. ( b ) PL decay dynamics of C/A/S QDs (total radius 7.0 nm; line 4 in Table 1 ) in solution (black), as a film on a glass substrate (blue), as a film on a ZnO/ITO substrate (green), and within a QD-LED at zero bias ( V =0) (red). Inset: PL lifetime for QDs within the device as a function of applied voltage ( V ≤ V on ). ( c ) Schematic illustration of QD charging in QD-LEDs under zero bias (upper panel) and under operational conditions ( V > V on ; lower panel). ( d ) Peak EQE and J 1/2EQE of QD-LEDs as a function of a relative PL QY of a negative-trion ( ). Full size image Spectroscopic signatures of QD charging in QD-LEDs To gain a better understanding of the physics underlying the operation of QD-LEDs, we studied the recombination processes within the QD layer of our devices using time-resolved PL spectroscopy ( Fig. 2b ). One striking observation is that the QDs within the LED, even without applied bias, show much faster PL decay compared with the same QDs in either a solution sample or in films assembled on a ‘passive’ glass slide. This observation cannot be attributed to mechanisms such as exciton quenching by energy transfer to CTLs because the QD band-gap ( E g =2.0 eV) is much smaller than that of the adjacent CTLs ( E g of ~3.3 eV for ZnO and 3.2 eV for CBP; Supplementary Fig. S2 ). Instead, a more feasible explanation is in terms of activation of Auger recombination due to electrons injected into the QDs from the cathode. Indeed the PL lifetime ( τ PL ) measured for the 7 nm C/A/S QDs within the devices is 8.6 ns, which is very close to the Auger recombination time of a negative-trion inferred from spectroscopic studies of QD solutions (~7 ns; Table 1 , line 4). We can rationalize these observations by considering the alignment of electronic states in different device layers. Specifically, for the inverted architecture used in our LEDs, the QD conduction-band level is located in energetic proximity to the Fermi level of the cathode, which can result in spontaneous (that is, at zero bias) electron injection into the QDs. On the other hand, hole injection is inhibited by a sizable energetic barrier in the valence band (almost equal to E g of the QDs), and therefore, it requires the assistance of an external electric field. This injection asymmetry can easily cause charging of the QDs with excess electrons even without bias, as well as under a small forward bias when the LED is operated in the low current-density regime ( Fig. 2c ). That the observed change in the QD PL decay upon incorporation into the devices is indeed due to excess electrons is confirmed by an analysis of variations in the PL lifetime under applied voltage (inset of Fig. 2b ). In the case of reverse bias, which makes electron injection less favourable, the PL decay actually becomes slower, as expected for the situation in which QDs fluctuating between the charged and the neutral states spend an increasing amount of time in the neutral state [29] . On the other hand, the PL dynamics get progressively faster under direct bias due to increasing contribution from doubly negatively charged excitons ( Fig. 2c ; lower panel) [29] . The above analysis suggests that during LED operation a significant fraction of the QDs in the emitting layer are negatively charged, and therefore the EL efficiency is likely more closely related to the PL QY of a negative-trion ( ) rather than of a neutral exciton ( Q X ). To characterize different samples used in this study in terms of their trion emission efficiency, we define a relative PL QY of X − as / Q X . Based on statistical arguments [30] , the purely radiative lifetime of a trion is twice as fast as that of a neutral exciton, and therefore, can be expressed via the measured (that is, total) τ X and lifetimes as / τ X . In the absence of Auger recombination, should be unity; however, because is essentially determined by Auger decay, it is much smaller. The actual value of is therefore a measure of how dramatically Auger recombination reduces the effective PL QY of the negative-trion relative to that of the neutral exciton, which is not affected by Auger decay. Using this expression, we find that is only about 5% in the C/S dots with the thinnest shell ( H =2 nm; Table 1 , line 1). As the shell thickness is increased, also increases (as a result of a reduced rate of Auger decay) and in dots with H =5.5 nm it approaches 20% ( Table 1 , line 3). A further increase in (up to 35%) occurs for QDs with an interfacial alloy layer introduced for additional suppression of Auger decay. Assuming a significant contribution from trions to EL, we might anticipate that the peak EQE will increase from sample 1 to 4, in correlation with the estimated values of . This is indeed observed in our experiments ( Table 1 ). As was pointed out earlier, single-exciton PL QYs show an opposite trend, suggesting once again the importance of emission from charged species in these LED devices. Efficiency roll-off and Auger recombination The degree of charging as well as the role of multicarrier non-radiative Auger recombination are expected to increase with increasing driving current, which is a likely reason for the observed EQE roll-off ( Fig. 2a ; see also Supplementary Fig. S4 ). This explanation is consistent with the fact that the onset of the roll-off ( J 1/2EQE ; defined here as the current-density at which the EQE drops by 50% from its peak value) shifts to higher currents for QDs with decreased rate of Auger recombination, and, respectively, increased emission QY of charged excitations ( Fig. 2d and Table 1 , compare rows 7 and 10). Some previous studies have suggested that in certain cases the EQE roll-off can be attributed to a reduction of the QD emission rate due to field-induced spatial separation between electrons and holes [20] , [21] . Our observations are inconsistent with this explanation, as it implies that CdSe/CdS QDs with thicker CdS shells should show a more dramatic decrease in the single-exciton PL QY as a function of applied bias, and therefore earlier EQE roll-off than samples with thinner shells, while we observe the opposite behaviour. Further, a distinct asymmetry in the effect of negative versus positive biases on PL lifetimes discussed earlier in this work (inset of Fig. 2b ) also argues against field-induced changes in carrier dynamics and EQEs, as the effect of an electric field should be independent of field direction. All of these considerations along with our experimental observations strongly suggest that the efficiency roll-off in our LEDs is due to an increasing degree of QD charging, which leads to enhanced carrier losses due to Auger recombination. A similar mechanism for the EQE roll-off has been previously shown to be operative in traditional LEDs based on epitaxial quantum-well emitters [18] , [19] . Consideration of the band-diagram of our LEDs along with the results of spectroscopic studies of carrier dynamics suggest that QDs in these devices are negatively charged under zero bias, and that the degree of negative charging further increases under forward bias. This is opposite to the assessment of a previous report by Mashford et al. [13] , which proposed that when QDs are brought in contact with a ZnO layer, they may acquire a net positive charge under zero bias, while application of increasing forward bias leads to restoration of charge balance (that is, charge neutrality) due to an increasing number of electrons injected into the emitting layer. Although this scenario seems consistent with their observations [13] , it is clearly not applicable to our devices. First of all, we observe a lengthening of PL lifetime indicative of QD ‘discharging’ not under forward but rather reverse bias ( Fig. 2b ; inset), which tends to remove electrons from the QDs. Further, using the measured X − and XX Auger time constants, we can estimate the X + lifetime from , which yields =2.2 ns for the C/A/S dots in Fig. 2b . This value is considerably shorter than the PL lifetime measured for these dots on the ITO/ZnO electrode (8.6 ns), while as was pointed out earlier, τ PL is close to the X − lifetime (7 ns). All of these points support our conclusion that the excess charges in the QDs within our devices are of negative sign. Signatures of multicarrier states in EL In addition to dynamical signatures of charging, we also see spectral signatures of multicarrier states in EL that become especially pronounced at high-current densities. In Fig. 3a,b , we compare devices based on C/S 3.5 nm and C/A/S 7.0 nm QDs that exhibit the greatest contrast with regard to emission efficiencies of charged species ( Table 1 , lines 1 and 4). QD-LEDs with the C/S QDs show a gradual EL spectral shift to lower energy with increasing current ( Fig. 3a ), in line with expectations for joule heating (see Supplementary Figs S5 and S6 that illustrate the effect of increasing temperature on PL of QD films). In sharp contrast, in QD-LEDs made of the C/A/S QDs, the EL shifts in the opposite direction, that is, to higher energies ( Fig. 3b ). This is a signature of increasing contribution from multicarrier emission. As was pointed out before, in core/shell CdSe/CdS QDs, electrons and holes are partially separated in space, which results in Coulombic repulsion in the case of multicarrier states [31] , [32] . As a result of this repulsion, the total energy of a multicarrier system is higher than the sum of energies of noninteracting carriers, which leads to a blue shift of the corresponding emission band [31] . 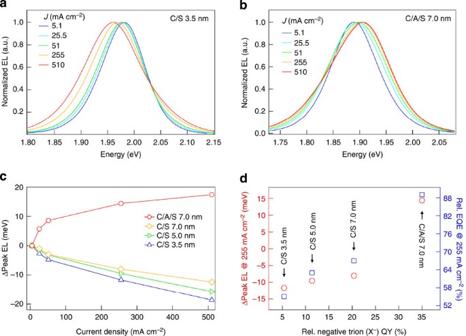Figure 3: Signatures of multicarrier states in electroluminescence spectra of QD-LEDs. Normalized EL spectra of QD-LEDs based on (a) C/S 3.5 nm and (b) C/A/S 7.0 nm under varied current densities. (c) EL peak shift in QD-LEDs with different types of QDs as a function of current-density. (d) EL peak shift (red circle) and relative EQE (blue square) of QD-LEDs at 255 mA cm−2as a function of relative PL QY of negative trions (). Figure 3: Signatures of multicarrier states in electroluminescence spectra of QD-LEDs. Normalized EL spectra of QD-LEDs based on ( a ) C/S 3.5 nm and ( b ) C/A/S 7.0 nm under varied current densities. ( c ) EL peak shift in QD-LEDs with different types of QDs as a function of current-density. ( d ) EL peak shift (red circle) and relative EQE (blue square) of QD-LEDs at 255 mA cm −2 as a function of relative PL QY of negative trions ( ). Full size image In a QD-LED, the competing trends from heating and Coulombic repulsion coexist; however, the relative contribution from the latter increases when the emission QY of multicarrier states is increased. The swing in the competition in favour of Coulomb repulsion with increasing efficiency of multicarrier emission is evident in Fig. 3c , in which we plot the EL spectral shift as a function of driving current for the C/S samples with different shell thicknesses along with the C/A/S sample. For the devices based on the C/S QDs, the EL shift is dominated by joule heating. However, its magnitude decreases with increasing shell thickness as a result of increasing contribution from multicarrier emission as the rate of Auger decay decreases (which can be correlated to an increased negative-trion QY, as in Fig. 3d ). For the C/A/S sample, the EL shift is of opposite sign, indicating that it is primarily due to Columbic repulsion; this suggests that LED emission at high currents is likely primarily due to multicarrier states. QD engineering for improved charge balance A clear additional step for achieving better performance in QD-LEDs is to improve the charge-injection balance within the QD active layer. One option would be to completely redesign the device architecture by changing the composition of the CTLs to alter the band alignments. However, a more practical approach that would allow us to retain the advantages of this proven combination of materials once again involves a subtle change in the QD structure. Specifically, to partially impede electron injection into the QD we have added a thin outer shell of Zn 0.5 Cd 0.5 S. In Fig. 4a , we compare QD-LEDs made of CdSe ( r =1.5 nm)/CdS ( H =0.5 nm)/Zn 0.5 Cd 0.5 S ( B =1.5 nm) (C/S/S, line 5 in Table 1 and Supplementary Fig. S7 ) QDs to devices based on reference C/S 3.5 nm QDs (line 1 in Table 1 ), which have the same overall size and similar optical properties (for example, PL QY of 80%, E g ≈1.95 eV, τ X =20 ns, τ XX =100 ps, and of 5%). The peak EQE of the QD-LED with C/S/S QDs reaches 7.5%, over eight times higher than the C/S device (0.9%). Moreover, the C/S/S LEDs demonstrate substantially improved roll-off behaviour with a J 1/2EQE of 970 mA cm −2 (as compared with 337 mA cm −2 ; Fig. 4a , lines 1 and 5 in Table 1 ). Importantly, spectroscopic analysis of QDs in devices shows that the PL decay of C/S/S QDs is not affected by applied bias ( Fig. 4b ), in contrast to a rapid shortening of PL lifetimes with increasing direct bias for reference QDs ( Fig. 2b ). Further, we observed that the PL lifetime (6–6.5 ns) is considerably longer than that of the negative-trion (0.5 ns), indicating that the Zn 0.5 Cd 0.5 S shell layer indeed suppresses QD charging, much in the same way that a similar shell has been shown to suppress photocharging [33] , resulting in significant improvements in both device efficiency and the roll-off characteristics. Importantly, these improvements were achieved without measurably affecting the turn-on voltage (2 V, as for dots without the Zn 0.5 Cd 0.5 S shell; Table 1 ), suggesting that even further enhancements may be attainable through refinement of these methods. 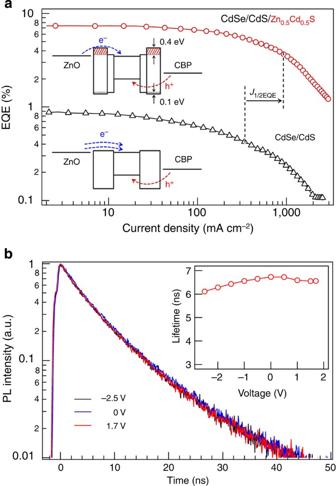Figure 4: QD-LEDs with improved charge balance through use of structurally engineered QDs. (a) EQE versus current-density of QD-LEDs with CdSe/CdS QDs (C/S 3.5 nm; lower inset and the trace shown by black triangles) and CdSe/CdS/Zn0.5Cd0.5S QDs (C/S/S 3.5 nm; upper inset and the trace shown by red circles). Vertical dashed lines indicate EQE roll-off onsets (J1/2EQE). (b) PL decay dynamics of C/S/S 3.5 nm QDs within a QD-LED under different applied biases (V<Von). Inset: PL decay lifetime of QDs within a QD-LED as a function of applied bias. Figure 4: QD-LEDs with improved charge balance through use of structurally engineered QDs. ( a ) EQE versus current-density of QD-LEDs with CdSe/CdS QDs (C/S 3.5 nm; lower inset and the trace shown by black triangles) and CdSe/CdS/Zn 0.5 Cd 0.5 S QDs (C/S/S 3.5 nm; upper inset and the trace shown by red circles). Vertical dashed lines indicate EQE roll-off onsets ( J 1/2EQE ). ( b ) PL decay dynamics of C/S/S 3.5 nm QDs within a QD-LED under different applied biases ( V < V on ). Inset: PL decay lifetime of QDs within a QD-LED as a function of applied bias. Full size image We have studied the role of multicarrier states and specifically the role of multicarrier Auger recombination in QD-LEDs. For these studies, we have utilized an inverted LED architecture, wherein a QD emitting layer is sandwiched between an inorganic, metal-oxide electron transport layer and an organic hole transport layer based on conjugated molecules. A key feature of this work is use of a series of structurally engineered heterostructured QDs in which the rate of Auger decay is systematically varied by either changing the shell thickness and/or by introducing an intermediate alloyed layer at the core/shell interface. Using these structures, we observe a direct correlation between the device performance and the rate of Auger decay. Specifically, LEDs based on C/A/S samples that exhibit the lowest rate of Auger recombination (and correspondingly the highest emission efficiencies of multicarrier states) show both the highest peak EQE as well as the highest threshold current for the onset of EQE roll-off. To rationalize these observations, we conduct spectroscopic studies of carrier dynamics in QDs within operational devices. We observe that even at zero bias the QDs are negatively charged, and the degree of charging increases under application of forward bias. This suggests that EL from these LEDs has a significant contribution from charged excitons and other multicarrier states of higher multiplicities, which leads to a significant impact of Auger on EQEs of these devices as well as the efficiency roll-off at high currents. These results suggest that further improvements in the performance of these devices should be possible by using dots with an even greater suppression of Auger decay and/or by applying measures that promote a more balanced injection of electrons and holes. In support of this latter assertion, we show that rational modification of the QD structure to incorporate an additional shell of a semiconductor with a higher conduction-band edge can improve the charge balance within the QDs by impeding electron injection, which leads to higher efficiency and better roll-off behaviour in devices. Ultimately, QD-LEDs for applications requiring very high brightness will likely need to apply both of these methods in concert, as the contributions from neutral multiexciton emission will become increasingly important at high-driving currents even if charge balance is strictly maintained. General materials considerations Cadmium oxide (CdO, 99.998%), Se (200 mesh, 99.999%), zinc acetate (Zn(Acet) 2 , 99.99%), S (power, 99%), 1-dodecanethiol (DDT, 98%), oleic acid (OA, 99%), 1-octadecene (ODE, 90%), tri-n-octylphosphine (TOP, 97%), tri-n-octylamine (TOA, 95%), zinc acetate dihydrate (Zn(Ac) 2 ·2H 2 O,>98%), potassium hydroxide (KOH, 99+%) and butanol (99%) were purchased from Alfa Aesar. Other organic solvents were purchased from Fisher Chemical. LD 690 perchlorate, used as a reference dye in PL QY measurements, was purchased from Exciton. All chemicals were used without further purification. All syntheses were performed under inert atmosphere using standard Schlenk-line and glovebox techniques. 0.5 M cadmium oleate [Cd(OA) 2 ] and zinc oleate [Zn(OA) 2 ] solutions were prepared by heating 5 mmol of CdO or Zn(Ac) 2 with 5 ml of OA at 300 °C for 1 h, and then diluting with TOA to a total volume of 10 ml. Trioctylphosphine selenium (1 M; TOPSe) or sulphur (TOPS) solutions were prepared by stirring 1 mmol of Se or S with 1 ml of TOP at room temperature overnight. Synthesis of CdSe/CdS and CdSe/CdSe 0.5 S 0.5 /CdS QDs Detailed synthesis and structural characterization was reported previously [22] . CdSe QDs with radius of 1.5 nm were synthesized by a previously reported method [34] . Prepared CdSe QDs were repeatedly purified by precipitating with ethanol and redispersing in toluene, and then dispersed in ODE at a concentration of 0.015 mM. For the synthesis of CdSe/CdSe 0.5 S 0.5 QDs, this CdSe core solution (2 ml) was added to a flask containing 8 ml of TOA and 0.6 ml of 0.5 M Cd(OA) 2 at 300 °C. A mixture of TOPSe (0.15 ml of 1 M solution) and DDT (0.15 mmol) diluted with TOA (total volume: 1 ml) was slowly injected into the reaction flask over 30 min. Aliquots were taken during the reaction for characterization. Fabrication of a CdS shell was carried out via continuous slow injection of Cd(OA) 2 (0.5 M) and DDT (0.5 M, diluted with TOA) at a rate of 2 ml per h into the reaction vessel containing either CdSe or CdSe/CdSe 0.5 S 0.5 QDs diluted with TOA (total volume: 10 ml). The reaction temperature was maintained at 300 °C throughout the formation of the complete CdS shell. Synthesized QDs were purified by repeated precipitation/redispersion using ethanol and hexane before further characterization. Synthesis of CdSe/CdS/Zn 0.5 Cd 0.5 S QDs Zn 0.5 Cd 0.5 S shell-growth was performed in the same reaction vessel used for CdSe/CdS QD synthesis without isolation or purification. In a typical synthesis, Zn(OA) 2 (2 ml, 0.5 M) and Cd(OA) 2 (1 ml, 0.5 M) were injected into the CdSe ( r =1.5 nm)/CdS ( H =0.5 nm) QD growth solution. TOPS (1 ml, 1 M) was then injected at 300 °C, and the reaction proceeded for 10 min. Product QDs were purified by repeated precipitation/dispersion using ethanol and hexane before further characterization. Synthesis of ZnO nanoparticles ZnO nanoparticles were synthesized via a modification of previously reported methods [35] . Zn(ac) 2 ·2H 2 O (3 g) and methanol (120 ml) were placed in 500 ml 3-neck round bottom flask and heated to 60 °C. At that temperature, KOH solution (1.51 g in 120 ml in methanol) was added dropwise. The reaction mixture was vigorously stirred at 60 °C for 135 min and then allowed to cool to room temperature. ZnO nanoparticles were collected by centrifugation at 4,000 r.p.m., and redispersed in 1-butanol (10 mg ml −1 ). Structural characterization The size and composition of QDs were characterized using a TEM (JEOL JEM 2010) equipped with an energy-dispersive X-ray (EDX) spectrometer (Bruker Quantax). TEM samples were prepared by drop-casting dilute sample solutions onto carbon-coated copper TEM grids. Spectroscopic characterization Optical absorbance was measured with an Agilent 8453 spectrometer; solution PL spectra and single-exciton decay traces were recorded with a Horiba Fluoromax-4 spectrofluorometer. The PL QYs were estimated by comparing their PL intensities with those of standard dye solutions (LD 690 from Exciton Corporation) at the same optical density (0.05) using the same excitation wavelength. Picosecond time-resolved PL measurements were conducted using a Hamamatsu 5860 streak camera with 12 ps time resolution. The samples were excited at 3.1 eV with 100 fs pulses from a 1-kHz amplified Ti:sapphire laser. In nanosecond PL measurements, the samples were excited at 3.1 eV by 250 fs pulses from a 250-kHz amplified Ti:sapphire laser and PL dynamics were resolved using time-correlated single-photon counting (TCSPC). These measurements utilized two types of detectors: a microchannel plate photomultiplier tube (PMT; time resolution 150 ps), used for samples with biexciton lifetimes longer than 300 ps, and a superconducting nanowire single photon detector (SNSPD) with the instrument response time of 50 ps in studies of samples with shorter biexciton decay times [36] . For microchannel plate detection, the collection monochromator was set to the PL peak wavelength while for SNSPD detection the PL was collected through a 610-nm long pass filter, which blocks any contribution of the shell emission. The SNSPD was housed in a closed-loop helium cryocooler and kept at 3.5 K. The superconducting nanowire of NbN was biased to ~90% of its superconducting critical current (typically 20 μA). The voltage pulses were amplified and read out with a Picoquant Hydraharp with an 8 ps binning time. Single-exciton radiative lifetimes were determined from monoexponential fits of the low-fluence (no multiexcitons) decay traces acquired with PMT-TCSPC, which yielded time constants of tens of nanoseconds. In these samples, non-radiative losses are primarily due to carrier trapping at surface/interfacial defects, which is characterized by much faster subnanosecond dynamics not resolvable in the PMT-TCSPC measurements. This approach to determining radiative time constants is validated by the fact that the single-exciton radiative lifetimes of our thin-shell samples are in good agreement with literature values for well-passivated core-only CdSe QDs. Statistical scaling of the radiative decay rates Using simple statistical arguments [30] , [37] , we assume that the radiative decay rate ( k m,rad ) of the multicarrier state scales linearly with the number of available recombination pathways, which is to say that it is proportional to the product of the number of electrons ( N e ) and the number of the holes ( N h ) within the multicarrier state. Then, k m,rad can be expressed as k m,rad = N e N h k X ,rad , where k X ,rad is the radiative decay rate of the neutral exciton. Therefore, for the negative trion with N e =2 and N h =1, we obtain k X − ,rad =2 k X,rad . Using this relation, the QY ratio between X − and X can be expressed as: Device fabrication and characterization All QDs were purified five times by sequential precipitation with ethanol and redispersion in hexane, followed by dilution to 15 mg ml −1 for device fabrication. QD-LEDs were fabricated on patterned ITO glass substrates, which were cleaned in an ultrasonic bath using isopropanol, acetone and methanol sequentially. ZnO layers were spin-cast from 1-butanol dispersions of ZnO nanoparticles onto cleaned ITO glass substrates at 2,000 r.p.m. and dried in an N 2 atmosphere at 90 °C for 30 min. QD active layers were then span-cast from dispersion at 4,000 r.p.m. CBP (Lumtec Corporation), MoO 3 and Al, respectively, were then sequentially deposited by thermal evaporation in a vacuum deposition chamber (1 × 10 −7 torr). The current–voltage–luminance characteristics were measured using a Keithley 236 source-measure unit and a Keithley 2,000 multimeter coupled with a calibrated Si photodiode. The EL spectra of the devices were obtained using a Konica-Minolta CS-1000 A spectroradiometer. Bias-voltage dependence of PL dynamics of QDs in devices was measured using TCSPC. Samples were excited with a 405 nm pulsed laser (~40 ps pulse width) at a repetition rate of 2 MHz, and photons emitted from QDs were recorded with a single photon detector (time resolution of~350 ps). How to cite this article: Bae, W. K. et al. Controlling the influence of Auger recombination on the performance of quantum-dot light-emitting diodes. Nat. Commun. 4:2661 doi: 10.1038/ncomms3661 (2013).